Imaging energy status in live cells with a fluorescent biosensor of the intracellular ATP-to-ADP ratio The ATP:ADP ratio is a critical parameter of cellular energy status that regulates many metabolic activities. Here we report an optimized genetically encoded fluorescent biosensor, PercevalHR, that senses the ATP:ADP ratio. PercevalHR is tuned to the range of intracellular ATP:ADP expected in mammalian cells, and it can be used with one- or two-photon microscopy in live samples. We use PercevalHR to visualize activity-dependent changes in ATP:ADP when neurons are exposed to multiple stimuli, demonstrating that it is a sensitive reporter of physiological changes in energy consumption and production. We also use PercevalHR to visualize intracellular ATP:ADP while simultaneously recording currents from ATP-sensitive potassium (K ATP ) channels in single cells, showing that PercevalHR enables the study of coordinated variation in ATP:ADP and K ATP channel open probability in intact cells. With its ability to monitor changes in cellular energetics within seconds, PercevalHR should be a versatile tool for metabolic research. The ATP:ADP ratio is a central control parameter of cellular energy metabolism that determines the free-energy change for ATP hydrolysis and therefore the driving force for many reactions [1] . In glucose metabolism, for example, the ATP:ADP ratio controls whether the reaction flux through phosphoglycerate kinase is in the glycolytic or gluconeogenic direction [1] . In other cases, the ATP:ADP ratio can exert control through allosteric regulation. In the citric acid cycle, for example, lowered ATP:ADP can stimulate substrate oxidation by isocitrate dehydrogenase [2] . Conversely, the ATP:ADP ratio is also a sensitive indicator of energy consumption and changes in cellular energy status [3] , [4] . Even mild stimulation of ATP hydrolysis can cause a large magnitude decrease in ATP:ADP because of the increase in [ADP], even if the change in [ATP] is small. Cellular energy status is important not only for cell health but also for regulating signalling activities. For example, the AMP-activated protein kinase (AMPK) monitors energy status by sensing changes in ATP:ADP in order to control the balance of catabolic and anabolic activities [5] , [6] . In general, whether through AMPK or other mechanisms, all cells integrate information about energy status and nutrient availability for regulating the metabolic activities that support their specific cell functions [3] , [5] , [6] . For instance, in electrically excitable cells such as neurons and neuroendocrine cells, metabolism and electrical signalling are coupled, and the dynamics of ATP:ADP can greatly influence signalling. When a neuron fires an action potential or receives synaptic input, ions such as Na + and K + move across the cell membrane. In order to restore resting ion gradients, ATP consumption is subsequently increased to support the ion pumping activity of the Na + /K + -ATPase [7] . As a consequence of these high-energy demands, neuronal signalling requires an efficient supply of fuel for ATP production; however, there are still many questions about how increased demand alters energy levels and how energy levels are maintained by increased production of ATP. Such metabolic management is important both for the survival of neurons in neurodegenerative diseases and for the control of their excitability [8] , [9] . One mechanism by which energy status exerts control over electrical excitability is through ATP-sensitive potassium channels (K ATP channels). The opening of K ATP channels is inhibited by ATP and stimulated by ADP [10] —in effect, responding to the ATP:ADP ratio. In resting pancreatic β cells, K ATP channels are normally open, but the increased supply of glucose after a meal elevates ATP:ADP, causing K ATP channels to close and the membrane to depolarize [11] . The substantial basal activity of K ATP channels remains somewhat puzzling: in excised membrane patches, K ATP channel opening is inhibited by ATP with a high-affinity inhibitory constant of 10 μM (refs 10 , 12 , 13 ), yet cytosolic ATP levels are 100 times higher [14] . Basal stimulation by ADP [15] , [16] , [17] , [18] , [19] or by the signalling lipid phosphatidylinositol-4,5-bisphosphate (PIP 2 ) could account for channel activity [17] , [20] , [21] , but study of the channels’ dose-response in intact cells, by simultaneous measurement of ATP:ADP and channel activity, is needed to resolve such questions. Real-time measurement of ATP:ADP ratios in intact cells requires an optical reporter because biochemical measurements are destructive and cannot achieve single-cell sensitivity. We previously reported the first fluorescent biosensor of ATP:ADP ratio, Perceval, but this sensor is not well tuned for use in mammalian cells [22] . Mammalian ATP:ADP ratios are expected to range from 1 to >100 under healthy conditions [1] , [14] , [23] , [24] , but Perceval saturates at low ATP:ADP ratios (ATP:ADP <5). This limits the effectiveness of Perceval, and an important goal has been to engineer a biosensor tuned to sense higher ATP:ADP values. To this end, we report an optimized biosensor, PercevalHR (Perceval High Range), that senses changes in the ATP:ADP ratios expected in healthy mammalian cells. PercevalHR visualizes ATP:ADP in live cells with single-cell resolution, it can be used with one- or two-photon excitation and it is spectrally compatible for multichannel imaging with other fluorescent sensors. To demonstrate that PercevalHR can sense physiological changes in energy status, we stimulate neurons and visualize reversible, activity-dependent changes in ATP:ADP that are not observed in astrocytes. We also image PercevalHR while recording K ATP single-channel activity in the cell-attached configuration, allowing us to directly correlate intracellular ATP:ADP with K ATP open probability in the same intact cell. Development of PercevalHR Using a structure-guided protein engineering strategy, we performed intensive mutagenesis on the amino-acid residues around the ATP-binding pocket of the original Perceval sensor [22] , [25] , [26] . After several cycles of screening, we obtained an improved variant, PercevalHR, that has an increased fluorescence response and senses a greater range of ATP:ADP ratios ( Supplementary Fig. S1 ). PercevalHR has a maximum signal change of more than eightfold for optimal wavelengths, a significant improvement compared with the maximum signal change of twofold for Perceval. The sensor has two distinct peaks in its excitation spectrum, at ~420 and ~500 nm, that respond differently to nucleotide binding ( Fig. 1 ). ATP binding increases the fluorescence for 500-nm excitation, whereas ADP increases the fluorescence for 420-nm excitation; there is a fixed isosbestic point at ~455 nm. The responses are primarily due to a change in the sensor’s absorbance ( Supplementary Table S1 ). By taking the ratio of the fluorescence at two different excitation wavelengths ( F high / F low or F high / F iso ), the ratiometric signal reports the occupancy of PercevalHR independent of the amount of sensor protein. 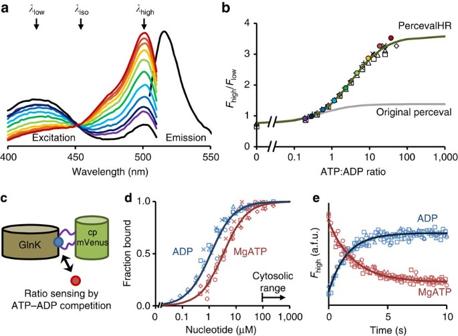Figure 1: PercevalHR sensor characterization. (a) Fluorescence excitation and emission spectra. Excitation spectra from blue to red indicate increasing ATP:ADP and correspond to the coloured data points in (b). (b) ATP:ADP dose-response of PercevalHR with Hill fit (green):KR=3.5±0.2;nH=0.97±0.04 (N=6). Scaled original Perceval response for comparison (grey)22. Dose-response curves and kinetics were obtained in constant 0.5 mM free Mg2+obtained by adjusting the total MgCl2concentration for the different nucleotide concentrations. See alsoSupplementary Fig. S2for detailed characterization of Mg2+-dependence. (c) Diagram of PercevalHR ATP:ADP sensing. (d) Binding curves for MgATP (red:Kapp=3.4±0.2 μM;nH=1.2±0.2;N=6; [MgATP] calculated) and ADP in the presence of EDTA (blue:Kapp=1.1±0.2 μM;nH=1.0±0.1;N=6). Expected range of cytosolic [ATP] and [ADP] is indicated14. (e) Apparent off rates for MgATP (red:τ=2.1±0.2 s;N=3) and ADP (blue:τ=1.5±0.1 s;N=3). Data are mean±s.e.m. Figure 1: PercevalHR sensor characterization. ( a ) Fluorescence excitation and emission spectra. Excitation spectra from blue to red indicate increasing ATP:ADP and correspond to the coloured data points in ( b ). ( b ) ATP:ADP dose-response of PercevalHR with Hill fit (green): K R =3.5±0.2; n H =0.97±0.04 ( N =6). Scaled original Perceval response for comparison (grey) [22] . Dose-response curves and kinetics were obtained in constant 0.5 mM free Mg 2+ obtained by adjusting the total MgCl 2 concentration for the different nucleotide concentrations. See also Supplementary Fig. S2 for detailed characterization of Mg 2+ -dependence. ( c ) Diagram of PercevalHR ATP:ADP sensing. ( d ) Binding curves for MgATP (red: K app =3.4±0.2 μM; n H =1.2±0.2; N =6; [MgATP] calculated) and ADP in the presence of EDTA (blue: K app =1.1±0.2 μM; n H =1.0±0.1; N =6). Expected range of cytosolic [ATP] and [ADP] is indicated [14] . ( e ) Apparent off rates for MgATP (red: τ =2.1±0.2 s; N =3) and ADP (blue: τ =1.5±0.1 s; N =3). Data are mean±s.e.m. Full size image The sensor binds nucleotides with very high affinity (1–3 μM; Fig. 1c,d ), and so at physiological concentrations it is always occupied by either ATP or ADP. Thus, when the sensor is expressed in cells, it is the ATP:ADP ratio rather than the absolute nucleotide concentrations that determines the fluorescence signal [22] . The ATP:ADP ratio at which PercevalHR shows a half-maximal signal change ( K R ) is ~3.5 with free [Mg 2+ ] of 0.5 mM, which is nearly seven times larger than the K R of ~0.5 for the original Perceval ( Fig. 1b ) [22] . Practically, PercevalHR senses ATP:ADP values from ~0.4 (10% sensor saturation) to 40 (92% sensor saturation), which is very well matched to the ATP:ADP range expected in mammalian cells. Time constants for ATP unloading and ADP unloading are ~2.1 and ~1.5 s, respectively, at 25 °C. Ligand-binding kinetics are typically faster at elevated temperature, and so we expect that the sensor can respond to changes in ATP:ADP ratio within a few seconds at room or physiological temperatures ( Fig. 1e ). PercevalHR responds specifically to the ATP:ADP ratio without significant interference from other metabolites such as α-ketoglutarate, AMP or GTP ( Supplementary Fig. S2 ). As discussed in the report for the original Perceval [22] , ATP binding is Mg 2+ -dependent, and free ATP does not induce an increase in signal ( Supplementary Fig. S2 ) [22] , [25] , [26] . PercevalHR exhibits pH-dependent sensing like many biosensors, but as previously demonstrated, we can approximately remove pH bias from true changes in ATP:ADP when imaging live cells [22] , [27] . We also validated that PercevalHR faithfully reports changes in intracellular ATP:ADP when expressed in live cells. In cultured neurons, metabolic inhibition caused a decrease in the sensor signal that was consistent with paired biochemical measurements of ATP:ADP using luciferase ( Fig. 2 ). The baseline signal and the change in signal caused by metabolic inhibition was independent of sensor concentration over a 10-fold range of expression levels, indicating that PercevalHR does not buffer ATP or ADP ( Fig. 2 ). 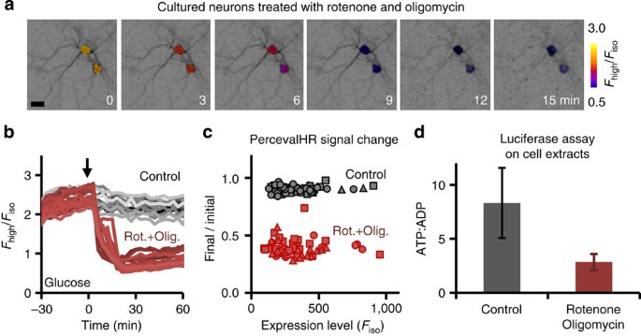Figure 2: PercevalHR reports changes in ATP:ADP in neurons. Cultured mouse embryonic cortical neurons imaged at 32±1 °C in glucose-containing solution were metabolically inhibited with 1 μM rotenone and 2.5 μM oligomycin. (a) Representative overlay images of two neurons. Background grayscale images show morphology. Foreground pseudocolored soma show the change in PercevalHR signal, reporting a decrease in ATP:ADP. Scale bar, 20 μm. (b) A representative experiment showing the time course of the PercevalHR ratiometric signal (Fhigh/Fiso) for individual neurons (grey, control, 17 cells; red, inhibitors, 20 cells; arrow, addition of vehicle control or inhibitors). Baseline signals and signal changes with metabolic inhibition are reproducible across cells. (c) The signal change of PercevalHR does not vary with expression level. The fluorescence intensity with excitation at the isosbestic point (xaxis,Fiso) is proportional to expression level. The signal change (yaxis) is the final PercevalHR ratiometric signal divided by the initial baseline signal. Data points in (c) correspond to the responses of individual cells shown in (b). (d) Subsequent to imaging, the same neurons in (a–c) were lysed, and the ATP:ADP was determined using a standard luciferase-based biochemical assay, verifying that ATP:ADP decreased for metabolically inhibited neuron cultures (n=3; mean±s.e.m.). Figure 2: PercevalHR reports changes in ATP:ADP in neurons. Cultured mouse embryonic cortical neurons imaged at 32±1 °C in glucose-containing solution were metabolically inhibited with 1 μM rotenone and 2.5 μM oligomycin. ( a ) Representative overlay images of two neurons. Background grayscale images show morphology. Foreground pseudocolored soma show the change in PercevalHR signal, reporting a decrease in ATP:ADP. Scale bar, 20 μm. ( b ) A representative experiment showing the time course of the PercevalHR ratiometric signal ( F high / F iso ) for individual neurons (grey, control, 17 cells; red, inhibitors, 20 cells; arrow, addition of vehicle control or inhibitors). Baseline signals and signal changes with metabolic inhibition are reproducible across cells. ( c ) The signal change of PercevalHR does not vary with expression level. The fluorescence intensity with excitation at the isosbestic point ( x axis, F iso ) is proportional to expression level. The signal change ( y axis) is the final PercevalHR ratiometric signal divided by the initial baseline signal. Data points in ( c ) correspond to the responses of individual cells shown in ( b ). ( d ) Subsequent to imaging, the same neurons in ( a – c ) were lysed, and the ATP:ADP was determined using a standard luciferase-based biochemical assay, verifying that ATP:ADP decreased for metabolically inhibited neuron cultures ( n =3; mean±s.e.m.). Full size image When expressed in Neuro2A neuroblastoma cells, PercevalHR also detected milder physiological changes in ATP:ADP that could not be detected by the original Perceval sensor. PercevalHR reported changes in ATP:ADP that were highly coupled to glucose supply, whereas the original Perceval sensor only detected a decrease in ATP:ADP caused by severe depletion of extracellular glucose ( Supplementary Fig. S3 ), demonstrating that PercevalHR is an important advance for monitoring physiological ATP:ADP dynamics. Imaging changes in ATP:ADP in astrocytes We next expressed PercevalHR in cultured astrocytes in order to investigate how acute changes in glucose supply affect cellular energy balance ( Fig. 3a ). It has not been clear to what extent astrocytes maintain ATP:ADP during glucose deprivation because biochemical measurements have been inconsistent, and nuclear magnetic resonance (NMR) measurements suggest that cell extraction introduces substantial artifacts [28] . To investigate this issue, we exposed PercevalHR-expressing astrocytes to different concentrations of extracellular glucose. We found that ATP:ADP in astrocytes could be tightly coupled to glucose supply; however, responses to changes in [glucose] and to metabolic inhibition were heterogeneous at the single-cell level ( Fig. 3 ; Supplementary Fig. S4 ). 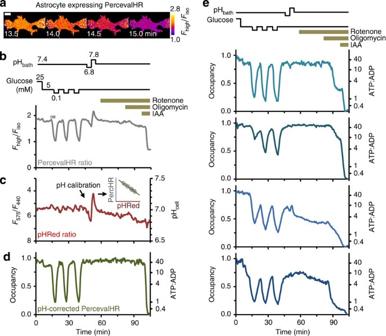Figure 3: Astrocyte ATP:ADP is coupled to extracellular glucose. (a) An astrocyte co-expressing PercevalHR and pHRed imaged at elevated temperature (31–34 °C). Image sequence shows the change in PercevalHR fluorescence ratio when [glucose] was lowered from 5 to 0.1 mM. Scale bar, 50 μm. (b) PercevalHR signal over time. Initial [glucose] was 25 mM, lowered to 5 mM, then lowered to 0.1 mM three times in sequence. Bath pH was varied from 6.8–7.8 for the pH calibration step following [glucose] changes. Rotenone, oligomycin and IAA were used at 1 μM, 2.5 μM and 1 mM, respectively. Vertical hash marks indicate approximate times for the images in (a). (c) pHRed fluorescence ratio (left axis). An absolute pH calibration was not necessary, but pH was estimated fromin vitrodata and shown for convenience only (right axis). Inset: from the pH calibration step, the empirical relationship between the PercevalHR signal and the pHRed signal shows a linear correlation describing the pH sensitivity of PercevalHR, which is used to approximately correct for pH bias. (d) PercevalHR sensor occupancy after approximate removal of pH bias (left axis) and the estimated ATP:ADP ratio (right axis). See alsoSupplementary Fig. S4. (e) Individual responses (after removal of pH bias) of four other astrocytes. Manipulations of [glucose] and pHbathas well as application of inhibitors was the same as described in (d). Figure 3: Astrocyte ATP:ADP is coupled to extracellular glucose. ( a ) An astrocyte co-expressing PercevalHR and pHRed imaged at elevated temperature (31–34 °C). Image sequence shows the change in PercevalHR fluorescence ratio when [glucose] was lowered from 5 to 0.1 mM. Scale bar, 50 μm. ( b ) PercevalHR signal over time. Initial [glucose] was 25 mM, lowered to 5 mM, then lowered to 0.1 mM three times in sequence. Bath pH was varied from 6.8–7.8 for the pH calibration step following [glucose] changes. Rotenone, oligomycin and IAA were used at 1 μM, 2.5 μM and 1 mM, respectively. Vertical hash marks indicate approximate times for the images in ( a ). ( c ) pHRed fluorescence ratio (left axis). An absolute pH calibration was not necessary, but pH was estimated from in vitro data and shown for convenience only (right axis). Inset: from the pH calibration step, the empirical relationship between the PercevalHR signal and the pHRed signal shows a linear correlation describing the pH sensitivity of PercevalHR, which is used to approximately correct for pH bias. ( d ) PercevalHR sensor occupancy after approximate removal of pH bias (left axis) and the estimated ATP:ADP ratio (right axis). See also Supplementary Fig. S4 . ( e ) Individual responses (after removal of pH bias) of four other astrocytes. Manipulations of [glucose] and pH bath as well as application of inhibitors was the same as described in ( d ). Full size image Figure 3 shows a representative response to [glucose] changes from a single astrocyte imaged at 31–34 °C. When [glucose] was lowered from 25 to 5 mM, a small decrease in the PercevalHR signal was observed ( Fig. 3b ). When [glucose] was further lowered to 0.1 mM, the PercevalHR signal decreased substantially and reversibly. After manipulating the extracellular [glucose], we subsequently added rotenone and oligomycin in sequence to block mitochondrial complex I and the ATP synthase, respectively. Rotenone caused a gradual decrease in the PercevalHR signal, whereas oligomycin caused a prompt small decrease. Lastly, the glycolytic inhibitor iodoacetic acid (IAA) was added, causing a large decrease in the PercevalHR signal. In this experiment, we co-expressed PercevalHR with the red fluorescent pH biosensor pHRed [27] . By concurrently imaging PercevalHR and pHRed, we observed that rotenone and oligomycin caused cellular acidification ( Fig. 3c ). Changes in pH can bias the PercevalHR signal, but this pH sensitivity can be corrected (Methods; Supplementary Fig. S4 ) [22] . Thus, in this and all cell-imaging experiments, we performed a calibration step allowing us to approximately remove pH bias, as previously reported ( Fig. 3c ; Methods; Supplementary Fig. S4 ) [27] . Furthermore, we normalize and present the pH-corrected PercevalHR signal in terms of the sensor occupancy ( Fig. 2d , left axis), which can be related to ATP:ADP assuming [Mg 2+ ] free ~0.5 mM ( Fig. 3d , right axis) [22] , [27] . After removing pH bias, it is evident that rotenone and oligomycin caused acidification but no appreciable change in ATP:ADP, suggesting that this astrocyte relied primarily on glycolysis for ATP production ( Fig. 3d ). Interestingly, we observed heterogeneity in responses to the mitochondrial inhibitors. Rotenone and oligomycin caused acidification in all cells, but after removal of pH bias it is clear that some astrocytes experience a decrease in ATP:ADP in response to both rotenone and oligomycin, whereas others responded only to oligomycin ( Fig. 3e ). Imaging activity-dependent energy consumption in neurons We also expressed PercevalHR in cultured neurons in order to investigate transient energy depletion caused by acute increases in neuronal activity. During and after stimulation of neurons, the movements of ions through channels leads to increased Na + /K + -ATPase ion pumping activity [29] , [30] . This increased hydrolysis of ATP and concomitant production of ADP should transiently decrease the ATP:ADP ratio [7] , [29] , [30] . To visualize transient activity-dependent energy consumption, we expressed PercevalHR and pHRed in dentate granule neurons cultured from postnatal mice. We compared the responses with three different stimuli (at 31–34 °C), presented sequentially: first, receptor activation with 50 μM glutamate for 6 s; second, membrane depolarization with 15 mM KCl for 30 s; and third, electrical stimulation with field electrodes (20 Hz, 250 pulses). The experiment shown in Fig. 4 illustrates differential ATP:ADP responses to the three stimuli as well as neuron-to-neuron heterogeneity in the responses. Activation of ionotropic glutamate receptors should cause an influx of sodium ions that greatly stimulates Na + /K + -ATPase activity, heavily consuming ATP. As expected, glutamate caused a large decrease in the ATP:ADP ratio that recovered slowly over several minutes ( Fig. 4a,b ). Both depolarization with KCl and stimulation with field electrodes cause activation of voltage-dependent channels (and potentially subsequent activation of synaptic channels), and these two stimuli caused smaller but clearly detectable decreases in ATP:ADP ratio that recovered rapidly ( Fig. 4b ). On average, glutamate stimulation caused a ~50±10% decrease in PercevalHR occupancy, while KCl and electrical stimulation caused ~30±10% and ~5±2% decreases in occupancy, respectively (mean±s.e.m. ; six experiments from independent cultures). 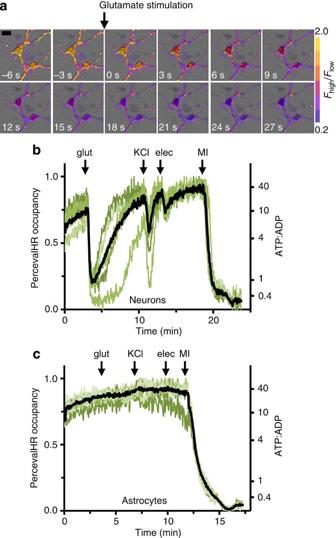Figure 4: Activity-dependent changes in neuronal ATP:ADP. (a) Cultured dentate granule neurons co-expressing PercevalHR and pHRed in a representative experiment conducted at elevated temperature (31–34 °C). Image sequence visualizes the change in PercevalHR fluorescence ratio with glutamate application. Scale bar, 20 μm. (b) Stimulation with 50 μM glutamate (glut), 15 mM KCl or field electrodes (elec; 20 Hz, 250 pulses) causes reversible decreases in ATP:ADP ratio. Metabolic inhibitors (MI: 1 mM IAA, 1 μM rotenone, 2.5 μM oligomycin) were added at the end of the experiment, and the pH calibration step was subsequently performed. Each green trace represents one neuron, the black trace represents the mean response (N=7 neurons in one representative experiment of 6). (c) Cultured astrocytes do not respond to the same stimuli (N=11 astrocytes). Figure 4: Activity-dependent changes in neuronal ATP:ADP. ( a ) Cultured dentate granule neurons co-expressing PercevalHR and pHRed in a representative experiment conducted at elevated temperature (31–34 °C). Image sequence visualizes the change in PercevalHR fluorescence ratio with glutamate application. Scale bar, 20 μm. ( b ) Stimulation with 50 μM glutamate (glut), 15 mM KCl or field electrodes (elec; 20 Hz, 250 pulses) causes reversible decreases in ATP:ADP ratio. Metabolic inhibitors (MI: 1 mM IAA, 1 μM rotenone, 2.5 μM oligomycin) were added at the end of the experiment, and the pH calibration step was subsequently performed. Each green trace represents one neuron, the black trace represents the mean response ( N =7 neurons in one representative experiment of 6). ( c ) Cultured astrocytes do not respond to the same stimuli ( N =11 astrocytes). Full size image We also expressed PercevalHR and pHRed in cultured astrocytes for comparison. In contrast to neurons, astrocytes did not respond noticeably to the same stimuli ( Fig. 4c ). Glutamate application was predicted to decrease the ATP:ADP ratio in astrocytes because uptake is coupled to Na + ion influx, and because increased glutamate metabolism through the glutamate–glutamine cycle should consume ATP [31] ; however, these data likely indicate that bathing in 50 μM glutamate is not a heavy metabolic burden for astrocytes in culture. Taken together, these results show that PercevalHR can easily detect physiological changes in ATP:ADP of different magnitudes and thus should be a broadly effective tool for investigating the coupling between metabolism and excitability. Correlating K ATP channel activity and ATP:ADP in intact cells The regulation of K ATP channel activity by ATP and ADP has been studied earlier by applying nucleotides to the intracellular face of membrane patches, physically excised from cells. To investigate how K ATP channels are regulated by energy status in intact cells, we imaged PercevalHR while simultaneously recording K ATP single-channel activity by patch-clamp in cell-attached mode at room temperature. PercevalHR and pHRed were co-expressed in HEK293 cells that stably express the Kir6.2 and SUR1 subunits of K ATP channels [32] , [33] . Cells were fed glucose, and then metabolically poisoned by either exchanging glucose for 2-deoxyglucose (2DG; Fig. 5 ) or by adding IAA ( Fig. 6 ). 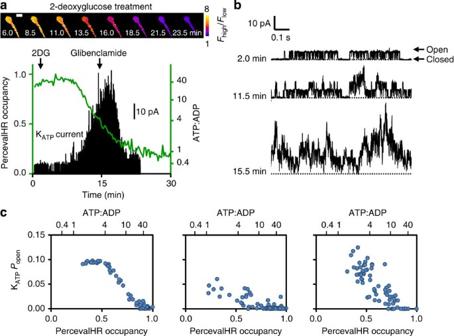Figure 5: Direct correlation of ATP:ADP and KATPsingle-channel activity in intact cells metabolically inhibited with 2-deoxyglucose. HEK293 cells expressing KATPchannels were recorded in 5 mM glucose at room temperature and then metabolically inhibited by the replacement of glucose with 10 mM 2DG. (a) Top image sequence visualizes the decrease in PercevalHR ratiometric signal with 2DG treatment for a single cell. Scale bar, 10 μm. Bottom panel shows that metabolic inhibition causes a decrease in ATP:ADP (green trace,yaxes) and a concomitant increase in KATPsingle-channel activity (black trace) for this cell. Channel activity was characteristic of KATPchannels and was inhibited by 200 nM glibenclamide33. (b) Examples of increasing single-channel activity. Inward currents are shown as upward deflections. (c) KATPsingle-channel open probability (Popen) versus PercevalHR occupancy shows thatPopenbegins to increase when ATP:ADP is ≥5. Left panel shows data from the same cell analysed in (a). Middle and right panels show data acquired from two other cells. See alsoSupplementary Fig. S5. Figure 5: Direct correlation of ATP:ADP and K ATP single-channel activity in intact cells metabolically inhibited with 2-deoxyglucose. HEK293 cells expressing K ATP channels were recorded in 5 mM glucose at room temperature and then metabolically inhibited by the replacement of glucose with 10 mM 2DG. ( a ) Top image sequence visualizes the decrease in PercevalHR ratiometric signal with 2DG treatment for a single cell. Scale bar, 10 μm. Bottom panel shows that metabolic inhibition causes a decrease in ATP:ADP (green trace, y axes) and a concomitant increase in K ATP single-channel activity (black trace) for this cell. Channel activity was characteristic of K ATP channels and was inhibited by 200 nM glibenclamide [33] . ( b ) Examples of increasing single-channel activity. Inward currents are shown as upward deflections. ( c ) K ATP single-channel open probability ( P open ) versus PercevalHR occupancy shows that P open begins to increase when ATP:ADP is ≥5. Left panel shows data from the same cell analysed in ( a ). Middle and right panels show data acquired from two other cells. See also Supplementary Fig. S5 . 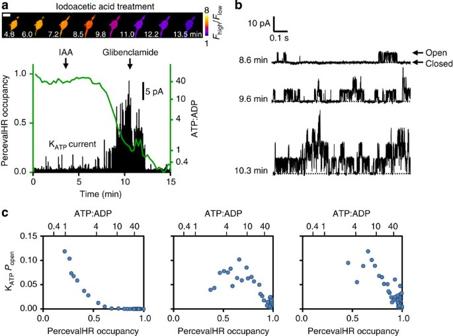Figure 6: Direct correlation of ATP:ADP and KATPsingle-channel activity in intact cells metabolically inhibited with iodoacetic acid. HEK293 cells expressing KATPchannels were recorded in 5 mM glucose at room temperature and then metabolically inhibited by supplementing with 1 mM IAA. (a) Top image sequence visualizes the decrease in PercevalHR ratiometric signal with IAA treatment for a single cell. Scale bar, 10 μm. Bottom panel shows that metabolic inhibition causes a decrease in ATP:ADP (green trace,yaxes) and a concomitant increase in KATPsingle-channel activity (black trace) for this cell. Channel activity was characteristic of KATPchannels and was inhibited by 200 nM glibenclamide33. (b) Examples of increasing single-channel activity. Inward currents are shown as upward deflections. (c) KATPsingle-channel open probability (Popen) versus PercevalHR occupancy shows thatPopenbegins to increase when ATP:ADP is ≥5. Left panel shows data from the same cell analysed in (a). Middle and right panels show data acquired from two other cells. See alsoSupplementary Fig. S6. Full size image Figure 6: Direct correlation of ATP:ADP and K ATP single-channel activity in intact cells metabolically inhibited with iodoacetic acid. HEK293 cells expressing K ATP channels were recorded in 5 mM glucose at room temperature and then metabolically inhibited by supplementing with 1 mM IAA. ( a ) Top image sequence visualizes the decrease in PercevalHR ratiometric signal with IAA treatment for a single cell. Scale bar, 10 μm. Bottom panel shows that metabolic inhibition causes a decrease in ATP:ADP (green trace, y axes) and a concomitant increase in K ATP single-channel activity (black trace) for this cell. Channel activity was characteristic of K ATP channels and was inhibited by 200 nM glibenclamide [33] . ( b ) Examples of increasing single-channel activity. Inward currents are shown as upward deflections. ( c ) K ATP single-channel open probability ( P open ) versus PercevalHR occupancy shows that P open begins to increase when ATP:ADP is ≥5. Left panel shows data from the same cell analysed in ( a ). Middle and right panels show data acquired from two other cells. See also Supplementary Fig. S6 . Full size image When glucose was exchanged for 2DG, PercevalHR reported a gradual decrease in intracellular ATP:ADP that was accompanied by increasing K ATP single-channel activity ( Fig. 5a ). At baseline, PercevalHR is saturated or near saturation, indicating basal ATP:ADP is ≥40 in these cells. Upon metabolic inhibition with 2DG or IAA, the PercevalHR signal decreased, reporting the expected decrease in intracellular ATP:ADP. The decrease in ATP:ADP occurred over several minutes, during which we observed multiple conductance levels corresponding to the activation of multiple channels in the recorded membrane patch ( Fig. 5b ). Thus, the increase in total current was a result of increased K ATP open probability ( P open ) and not a change in single-channel conductance. After K ATP activity increased substantially, we confirmed that the single-channel activity could be inhibited with the sulfonylurea drug glibenclamide at 200 nM, verifying that the observed currents originated from K ATP channel openings [33] . Similar to 2DG treatment, IAA caused a decrease in intracellular ATP:ADP that was accompanied by an increase in K ATP single-channel activity ( Fig. 6 ). In this case, IAA caused a faster decrease in ATP:ADP compared with 2DG treatment. As a result, K ATP channel activity also increased more rapidly when IAA was used. We cannot make firm conclusions about biological differences between 2DG and IAA inhibition kinetics because here perfusion and mixing kinetics confound the interpretation. These experiments clearly demonstrate that PercevalHR enables changes in K ATP channel activity to be directly correlated with changes in cytosolic ATP:ADP in intact cells. Upon examination of K ATP single-channel P open versus PercevalHR occupancy, it is evident that a similar correlation exists when either 2DG ( Fig. 5 ) or IAA ( Fig. 6 ) was used ( Supplementary Figs S5 and S6 ). The single-channel P open takes into account the number of channels in the patch so that this correlation is representative of the intrinsic coupling between ATP:ADP and K ATP channel activity. Taken together, metabolic inhibition caused an increase in the K ATP channel P open that was initially observed when ATP:ADP was only reduced to ratios of 5 to >10, still high-energy values ( N =6 cells; Figs 5 and 6 ; Supplementary Figs S5 and S6 ). Furthermore, K ATP channel activity reached the expected near-maximal P open ≈0.1 for intact cells [19] at ATP:ADP ratios of 1–4, before cells are expected to be in a state of severe energy crisis ( N =6 cells; Figs 5 and 6 ; Supplementary Figs S5 and S6 ). Imaging PercevalHR with two-photon excitation PercevalHR can also be used with two-photon excitation, which is valuable for measuring cellular energy status in thick samples such as tissue slices. Although two-photon excitation does not in general produce spectra corresponding exactly to the doubled one-photon excitation spectra [34] , we found that purified PercevalHR protein exhibits distinct two-photon excitation spectra in the ATP- and ADP-loaded states ( Fig. 7a ). We confirmed that it can indeed be ratiometrically monitored using two-photon imaging of PercevalHR and pHRed expressed in HEK293 cells. We simultaneously collected green fluorescence emission from PercevalHR in one detector channel and red fluorescence emission from pHRed in a second detector channel ( Fig. 7b ). In this experiment, we monitored intracellular pH with pHRed in fluorescence lifetime mode, using two-photon excitation at 840 nm ( Fig. 7b , top panels) [27] . The PercevalHR fluorescence ratio, monitored with two-photon excitation at 950 nm and 840 nm, reported a clear reduction in ATP:ADP upon metabolic inhibition ( Fig. 7b (bottom panels) ). As expected, this change was accompanied by slow cellular acidification, as seen in the one-photon imaging experiments ( Fig. 7c ). 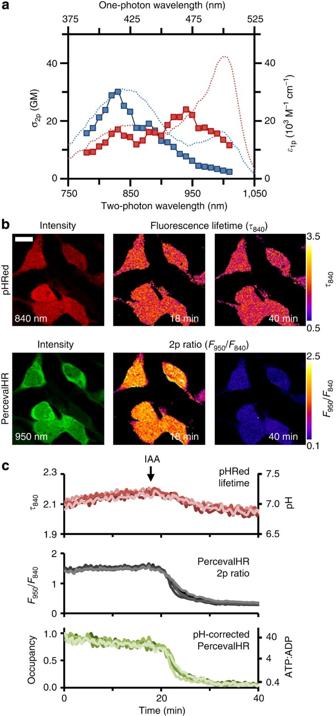Figure 7: Ratiometric imaging of PercevalHR with two-photon excitation. (a) Two-photon absorption cross section (σ2p) of PercevalHR protein (squares; left and bottom axes). One-photon absorption spectra (ε1p) shown for reference (dotted lines; right and top axes). ADP-loaded in the presence of EDTA (blue) and MgATP-loaded in the presence of excess Mg2+(red). (b) HEK293 cells co-expressing PercevalHR (bottom) and pHRed (top) were imaged in 5 mM glucose at room temperature. Scale bar, 20 μm. Left, fluorescence intensity images with two-photon excitation. Middle, high ATP:ADP state. Middle bottom, PercevalHR ratio with two-photon excitation at 950 nm and 840 nm. Middle top, pHRed lifetime with 840 nm two-photon excitation. Right, after metabolic inhibition with 1 mM IAA. (c) PercevalHR, pHRed and pH-corrected PercevalHR occupancy show that inhibition of glycolysis with IAA causes a large decrease in ATP:ADP ratio. Traces in (c) correspond to the five cells shown in (b). Figure 7: Ratiometric imaging of PercevalHR with two-photon excitation. ( a ) Two-photon absorption cross section ( σ 2p ) of PercevalHR protein (squares; left and bottom axes). One-photon absorption spectra ( ε 1p ) shown for reference (dotted lines; right and top axes). ADP-loaded in the presence of EDTA (blue) and MgATP-loaded in the presence of excess Mg 2+ (red). ( b ) HEK293 cells co-expressing PercevalHR (bottom) and pHRed (top) were imaged in 5 mM glucose at room temperature. Scale bar, 20 μm. Left, fluorescence intensity images with two-photon excitation. Middle, high ATP:ADP state. Middle bottom, PercevalHR ratio with two-photon excitation at 950 nm and 840 nm. Middle top, pHRed lifetime with 840 nm two-photon excitation. Right, after metabolic inhibition with 1 mM IAA. ( c ) PercevalHR, pHRed and pH-corrected PercevalHR occupancy show that inhibition of glycolysis with IAA causes a large decrease in ATP:ADP ratio. Traces in ( c ) correspond to the five cells shown in ( b ). Full size image PercevalHR is a broadly useful and faithful reporter of intracellular ATP:ADP, as seen from its ability to visualize energy changes in live Neuro2A neuroblastoma cells, primary astrocytes, primary neurons and HEK293 cells. The development of PercevalHR is an important technical advance because the original Perceval sensor was tuned to sense changes in ATP:ADP ratios upon extreme metabolic inhibition, but did not function in the more physiological range of ATP:ADP>5 expected in healthy mammalian cells. We directly compared the performance of the two sensors in Neuro2A cells, and found that only PercevalHR was highly sensitive to physiological energy changes. This important advance was achieved by shifting the sensor K R as well as increasing the signal dynamic range through structure-guided protein engineering. PercevalHR has a much larger magnitude fluorescence signal change, and its brightness is similar to other circularly permuted fluorescent protein sensors [35] , [36] . Compared with current methods used for monitoring ATP:ADP ratios, PercevalHR is a significant improvement in several regards. Current biochemical methods provide population-averaged measurements from cell extracts, but cell extraction can introduce significant errors in measurements [28] . Cell extraction releases total nucleotide content, confounding cytosolic and mitochondrial energy status; further, because much if not most of the ADP pool is protein-bound [24] , standard biochemical measurements underestimate ATP:ADP for the free nucleotides [1] . An alternate, noninvasive method, 31 P-NMR, can facilitate tissue and in vivo measurements of free ATP and ADP; however, NMR is relatively insensitive and lacks single-cell spatial resolution [37] . Luminescence imaging of single cells expressing luciferase has been used to monitor cellular energy status [38] ; however, image acquisition times are typically long (tens of seconds), and luciferase consumes ATP. In contrast, PercevalHR can continuously report ATP:ADP ratios for the non-bound nucleotides in single, intact cells with a time resolution of seconds. The PercevalHR signal is also a spectral ratio, which is important for live-cell imaging because this readout is intrinsically normalized, eliminating signal variation due to sensor expression levels and minimizing signal drift due to photobleaching. Furthermore, we demonstrated that PercevalHR can be imaged with either one-photon or two-photon excitation, making it a versatile tool for monitoring ATP:ADP dynamics in a wide variety of living samples and in a cell-specific manner, even in samples containing mixed cell populations. By expressing PercevalHR in cultured primary astrocytes, we were able to monitor coupling between extracellular [glucose] and the intracellular ATP:ADP. As this approach provided single-cell resolution, we were able to visualize heterogeneity in astrocyte energy metabolism. We observed general responsiveness to changes in [glucose], but we also observed varying sensitivity to the mitochondrial inhibitors rotenone and oligomycin, indicating that PercevalHR could be a useful reporter for investigating mitochondrial function. We also demonstrated that PercevalHR is spectrally compatible with red fluorescent proteins, allowing us to co-express the red pH biosensor pHRed for cell-by-cell correction of pH bias. Many fluorescent proteins [39] and biosensors like PercevalHR are pH-sensitive, including the gCaMP and GECO calcium sensors [40] , [41] , the HyPer hydrogen peroxide sensor [42] , and the iGluSnFR glutamate sensor [43] . Ideally, biosensors would be pH-insensitive [44] ; however, this is not trivial to engineer. Thus, because physiological and pathological changes in intracellular pH are common [45] , [46] , care must be taken to avoid misinterpretation of the reporter response [47] . We consistently observed that metabolic inhibitors caused cellular acidification, and we similarly observed that neuronal stimulation caused cellular acidification proportional to the strength of the stimulus. These manipulations produced changes of <0.5 pH units, often mild shifts of ≤0.1 pH units; however, for pH-sensitive probes these changes could still generate pH bias in their readout, and a pure change in pH could masquerade as a sensor signal. Therefore, we applied a simple calibration strategy that we previously reported for the approximate removal of pH bias from biosensor signals on a cell-by-cell basis [22] , [27] . Cell-to-cell variability in metabolic responses can be large even in cultured cell lines [48] . Thus, removing pH bias on a cell-to-cell basis is much more robust and reliable than comparing population averages from parallel experiments. Furthermore, our approach has the added benefit of collecting intracellular pH data, which itself may be interesting and important [49] , [50] . We next showed in neurons that PercevalHR can sense transient energy changes over a wide range of magnitudes, on physiologically relevant time scales. Activity-dependent changes in ATP consumption and production are fundamental to brain energy metabolism, and they ultimately underlie the processes governing clinically relevant PET and fMRI signals [51] . Many questions remain about brain fuel utilization and in particular metabolic coupling between neurons and astrocytes [8] , and we demonstrated here that PercevalHR should be an effective tool to investigate molecular and cellular metabolic processes. A strength of live-cell imaging is its compatibility with other methodology such as electrophysiology. To demonstrate the effectiveness of imaging of PercevalHR during electrophysiological experiments, we simultaneously tracked intracellular ATP:ADP while recording K ATP single-channel activity in intact cells. This work is an important step forward for K ATP channel physiology because PercevalHR should allow the relationship between cellular energy status and channel behaviour to be defined with greater detail. It has been proposed that in the cellular environment, hydrolytic activity of the SUR1 subunit or other ATPases supports the production of stimulatory ADP, allowing channels to be far more active in intact [15] or permeabilized β-cells compared with excised patches [19] . In metabolically inhibited HEK293 cells, we observed K ATP channels could be activated when cytosolic ATP:ADP was still high (>5). Theoretically, at an ATP:ADP ratio of 5, assuming a pool size of 4 mM (ref. 14 ) and an adenylate kinase equilibrium constant of ~1 (ref. 1 ), the concentrations of ADP and ATP are ~0.6 mM and ~3.2 mM, respectively. ADP concentrations of 0.1–0.2 mM have been shown to shift the apparent K i for ATP from 0.01 to 0.1 mM (refs 15 , 17 , 19 ). It is possible that our observations are explained by an ADP stimulatory effect in intact cells; however, the high ATP level might still be expected to keep K ATP channels closed [15] , [19] . Alternatively, basal PIP 2 levels in these cells could be high. PIP 2 dramatically decreases the sensitivity of the channel to ATP inhibition [20] , [21] , and thus high PIP 2 levels could allow K ATP channels to respond to changes in ATP:ADP ratios >5 (ref. 18 ). Clearly, these proof-of-concept experiments demonstrate that PercevalHR provides a methodology to more fully explore this issue and to learn details of K ATP physiology in intact cells. In conclusion, we have developed an optimized biosensor, PercevalHR, that senses changes in ATP:ADP over a large physiological range and can be used to visualize energy changes in living cells. The study of cellular energy metabolism relies on the technologies available to observe and measure intracellular ATP, ADP and AMP. Although biosensors for ADP and AMP are not yet available, PercevalHR reports related information about these metabolites. A critical distinguishing feature of PercevalHR is that it is sensitive to changes in ATP:ADP but not to changes in the total adenine nucleotide pool size. An alternative for sensing [ATP] directly, the ATeam biosensor, has also been reported [52] . For ATP-dependent reactions, ATP:ADP is a determinant of reversibility and driving force, whereas total ATP is a determinant of reaction rate and total turnover capacity. Although these two parameters are closely related, studies using ATeam have demonstrated that they can vary independently and changes in ATP level can be entangled with changes in the total nucleotide pool size, obscuring changes in ATP:ADP [53] . Thus, it will be particularly interesting in the future to use both PercevalHR and ATeam to dissect the distinct metabolic consequences of changes in ATP:ADP and total ATP level. Therefore, PercevalHR will enable new questions to be addressed concerning the dynamics of adenine nucleotides in cellular energy metabolism. Materials Unless otherwise indicated, all chemicals were purchased from Sigma, cell culture reagents were purchased from Invitrogen and optical filters were from Semrock. Molecular biology and protein screening PercevalHR was developed by mutating the original Perceval sensor at and around the GlnK nucleotide-binding site. Intensive mutagenesis was performed by a PCR strategy with mutagenic oligonucleotide primers containing codon variation introduced by using nucleotide mixtures during oligonucleotide synthesis (Alpha DNA). Error-prone PCR was conducted with a commercial kit (Stratagene). Mutagenized genes were cloned into the pRsetB (Invitrogen) bacterial expression vector providing an N-terminal His 7 tag and transformed into DH5α Escherichia coli. Single transformants were grown in YT media with 100 μg ml −1 carbenicillin selection in 96-well format (deep-well, 1.5 ml culture volume) overnight at 37 °C and then transferred to room temperature for 2–3 days additional growth. We found that leaky expression at room temperature was sufficient for screening purposes, and induction using BL21 or a similar strain was not necessary. Bacteria were pelleted by centrifugation, pellets were lysed with assay buffer (in mM: 100 MOPS, 50 KCl, 5 NaCl, 0.5 MgCl 2 ; pH 7.4) containing CellLyticB (Sigma) and crude lysates were transferred to nickel-coated 96-well plates overnight at room temperature to capture protein (HIS Select, Sigma). Capture plates containing protein were washed three times with phosphate-buffered saline containing 0.1% Tween-20 and three times with assay buffer. Purified protein was eluted from the plates with assay buffer containing 20 mM imidazole and 0.1% bovine serum albumin (BSA) and transferred to 96-well plates pre-blocked with assay buffer containing 0.1% BSA. Purified protein characteristics were screened in a fluorescence microplate reader (Synergy 4, BioTek) with additions of ADP and ATP holding free magnesium constant at 0.5 mM to construct a dose-response curve. For large-scale protein production, protein was expressed in 150–200 ml bacterial cultures and purified by nickel-affinity low-pressure chromatography (HiTrap Chelating HP, 1 ml bed volume, GE Lifesciences). Solutions were based on the manufacturer’s recommendations (Buffer A, in mM: 25 sodium phosphate; 500 NaCl; 10 imidazole; 5% glycerol; pH 7.5) with modifications as indicated, and chromatography was conducted at a flow rate of 0.8 ml per min. Cell pellets were collected by centrifugation, lysed with three freeze–thaw cycles followed by 15 min of agitation at room temperature in Buffer A supplemented with 2 × CellLyticB (Sigma), 1 mM dithiothreitol (DTT), 1 mM phenylmethanesulfonylfluoride (PMSF) and benzonase (Novagen). Lysate was cleared by centrifugation at >15,000 g for 10 min at 4 °C. The metal affinity column was charged with nickel and washed per manufacturer’s instructions. The nickel-charged column was equilibrated with 10 column volumes of Buffer A supplemented with 2 × CellLyticB before loading the cleared lysate. The loaded column was washed with 10 column volumes of Buffer B (Buffer A plus 1 × CellLyticB and final 20 mM imidazole) and 10 column volumes of Buffer C (Buffer A plus final 20 mM imidazole). Protein was eluted with Buffer D (Buffer A plus final 150 mM imidazole), collecting 0.2 ml eluate fractions. Fractions with highest fluorescence were pooled and dialyzed overnight at 4 °C in the dark against storage buffer (5 mM MOPS, 300 mM NaCl, 10% glycerol, pH 7.3) with three buffer changes. Protein concentration was determined by the BCA method (Pierce) and from denatured chromophore absorbance (NanoDrop, ThermoScientific), and aliquots were flash frozen and stored at −80 °C. Protein samples were still functional after >1-year storage. Additional fluorescence characterization was performed with a cuvette spectrofluorometer (Horiba), and kinetic measurements were performed with a manual rapid-mixing device (RX.2000, Applied Photophysics). Dose-responses and sensor kinetics were performed in the presence of 0.5 mM free Mg 2+ by adjusting the total MgCl 2 concentration for the different nucleotide concentrations. Calculation of [MgATP], [MgADP], [free ATP] and [free ADP] were performed with WebmaxC ( www.stanford.edu/~cpatton/webmaxcE.htm ) Plasmids encoding PercevalHR have been deposited with and are distributed through Addgene. Cell culture Maintenance of HEK293 cells stably expressing Kir6.2 and SUR1 has been previously described [32] , and these cells were used for all experiments involving HEK293 cells. Briefly, cells were maintained in MEM supplemented with 10% FBS, 300 μg ml −1 Zeocin and 700 μg ml −1 G418. For imaging, cells were plated on glass pre-coated in 1 mg ml −1 protamine. Stable cells were transfected with plasmids encoding PercevalHR and pHRed (Effectene, Qiagen) or transduced with lentivirus at a multiplicity of infection of 20. PercevalHR and pHRed were cloned into lentivirus vectors with the human Ubiquitin C promoter, and the virus was produced at the Massachusetts General Hospital viral core. Astrocyte cultures were made from P0–P4 mice and maintained in DMEM/F12 supplemented with 10% FBS. Neuron cultures were made from isolated cortices or hippocampi from E16–E18 mice or from isolated dentate gyrus from P15 mice (Charles River, C57BL/6N). Neurons were plated on glass that had been cleaned with nitric acid and pre-coated with poly- D -lysine. Cultures were maintained in Neurobasal-A (without glucose, Invitrogen) supplemented with 5–25 mM glucose, 0.2 mM pyruvate, 0.5 mM GlutaMax (Invitrogen), B-27 (Invitrogen), penicillin, streptomycin and used from 7–14 days in vitro with 50% feedings every 3–4 days. Cultured neurons were transfected with the calcium phosphate method [54] or infected with lentivirus at a multiplicity of infection of ~5. Animal procedures were approved by and performed in accordance with guidelines by the Harvard Institutional Animal Care and Use Committee. Live-cell fluorescence microscopy Cells were imaged on a Nikon TiE inverted microscope equipped with an Andor Revolution DSD spinning disk unit using a × 20/0.75 N.A. objective illuminated with an LED light source (Lumencor, Spectra X). PercevalHR was excited using 482/18 and 445/20 nm band-pass filters, emission was collected through a 529/39 nm band-pass filter, and excitation and emission light was separated with a 490-nm short pass dichroic. pHRed was excited using 578/16 and 445/20 nm band-pass filters, emission was collected through a 629/56 nm band-pass filter and a 590-nm short pass dichroic was used. Neurons were imaged in a home-built stimulation chamber using platinum–iridium foil field electrodes connected to a field stimulation unit. Neurons and astrocytes were continuously perfused at ~2 ml min −1 with bath solution heated to ~31–34 °C containing, in mM: 120 NaCl, 3 KCl, 2 CaCl 2 , 1MgCl 2 , 3 NaHCO 3 , 1.25 NaH 2 PO 4 , 15 HEPES, 5 glucose, 0.2 pyruvate, 0.5 GlutaMax (pH 7.4). Approximate removal of pH bias was performed as previously described [27] . Intracellular pH was varied by changing extracellular pH or by applying a standard 5–15 mM NH 4 Cl (ref. 55 ), and this calibration was performed over a short time period to minimize metabolic stress on the cell, maintaining an approximately constant ATP:ADP despite the changing pH [56] , [57] . Briefly, an empirical linear correlation between the uncorrected PercevalHR signal and pHRed signal was established using data collected during the calibration period. The relationship was used to predict pH bias in the PercevalHR signal over the entire experiment using the pHRed signal, and the uncorrected PercevalHR was normalized to approximately correct for the predicted pH bias ( Supplementary Fig. S4 ). The pH-corrected PercevalHR signal could be further transformed to a sensor occupancy because in all experiments calibration points for the ATP-saturated and ADP-saturated were estimated from high glucose and fully metabolic inhibited end points [22] , [27] . Luciferase assay Mouse embryonic cortical neurons were plated on glass-bottom 24-well plates (cleaned with nitric acid and pre-coated with poly- D -lysine). Assay solution contained B-27, essential amino acids (Invitrogen), and in mM: 10 glucose, 100 NaCl, 5.33 KCl, 1.8 CaCl 2 , 0.814 MgCl 2 , 0.906 NaH 2 PO 4 , 26.19 NaHCO 3 , 10.92 HEPES, 0.5 GlutaMax, 0.4 glycine, 0.4 serine (pH 7.4). Rotenone and oligomycin were used at 1 and 2.5 μM final concentrations, respectively. Neurons were imaged in a stage-top incubator heated to 32±1 °C with constant headspace flow of a humidified 5% CO 2 /95% air gas mixture. Neurons were imaged for 30 min for baseline measurements, then vehicle control or inhibitors were added, and neurons were imaged for an additional hour. After imaging, cells were immediately lysed, and ATP levels were quantified with a commercial luciferase kit (ATPLite, Perkin-Elmer) using a standard curve. To quantify ATP plus ADP, ADP in the extracts was converted to ATP with pyruvate kinase and phosphoenolpyruvate. Simultaneous imaging and electrophysiology Dual imaging and electrophysiology experiments were conducted on an Olympus BX51WI upright microscope using a × 40/0.80 water immersion objective. PercevalHR was excited using a Xenon lamp and monochromator (TILL Photonics, Polychrome IV) at 485 and 408 nm, and pHRed was excited at 575 and 485 nm. A triple-band dichroic was used (69002, Chroma) to separate emission light that was collected with a CCD camera (TILL Photonics, IMAGO-QE) using a dual-view image splitter (Optical Insights) with 529/24 and 629/53 nm band-pass filters. Cell-attached patch recordings were made in voltage-clamp mode (pipette voltage held at 0 mV) following establishment of high-resistance (multi-GΩ) seals. Data were acquired with a HEKA EPC 10 patch-clamp amplifier using Patchmaster v2 × 53 software (HEKA Instruments Inc.). Single-channel currents were filtered at 1 kHz and sampled at 5 kHz. All recordings were obtained at room temperature. Patch pipettes were pulled from borosilicate glass (Warner Instruments) and fire-polished to resistances of 3–5 MΩ when filled with recording solutions. The pipette solution contained (in mM): 140 KCl, 2.6 CaCl 2 , 1.2 MgCl 2 , 5 HEPES (pH to 7.4 with KOH) and the bath solution: 140 NaCl, 2.5 KCl, 2 CaCl 2 , 1 MgCl 2 , 10 HEPES (pH to 7.4 with NaOH). Recordings were made in 5 mM external glucose with continuous perfusion of bath solution. IAA was used at 1 mM final concentration in the 5 mM glucose bath solution. 2DG was used at 10 mM with no additional glucose. Glibenclamide was used at 200 nM, diluted in bath solution from a 200 mM stock solution in DMSO. NH 4 Cl (15 mM) was used for the pH calibration, diluted in bath solution from a 1 M stock solution in water. Single-channel analysis was performed using QuB ( www.qub.buffalo.edu ) and Matlab (Mathworks). Open and closed levels for channel activity were detected using a 50% threshold criterion. Raw data sets featuring excessive baseline shift or sufficient high- or low-frequency noise to preclude effective idealization of channel openings were discarded. The number of channels in the patch was estimated from the maximum number of simultaneous channel openings observed, which agreed with binomial analysis and method of moments estimator. Two-photon excitation fluorescence microscopy Two-photon excitation fluorescence protein characterization and live-cell microscopy were performed on the same imaging station essentially as previously described [27] with modifications. An upright microscope with × 60/0.90 N.A. water immersion objective (Olympus, BX51WI) was modified for two-photon excitation fluorescence microscopy and two-photon excitation fluorescence lifetime imaging microscopy by R.M., G.Y., Yao Chen and Bernardo Sabatini. Samples were excited using a tunable Ti:Sapphire 80 MHz laser (Coherent, Chameleon Vision II). Integrated photon counts for PercevalHR fluorescence and fluorescence decays for pHRed were measured using a time-correlated single-photon counting board (Becker and Hickl SPC-150). Fluorescence emission of the two sensors was collected simultaneously with two photomultiplier tubes (Hamamatsu H7422). PercevalHR fluorescence emission was collected using a 525/50 nm band-pass filter, and pHRed fluorescence emission was collected using a 630/60 nm band-pass filter. The two-photon absorption cross-section of purified PercevalHR protein was measured relative to fluorescein [34] , [58] , and live-cell imaging experiments were performed essentially as described above. Data were collected and analysed using Matlab software provided by Bernardo Sabatini and modified for lifetime imaging microscopy by G.Y., based partly on code provided by Ryohei Yasuda. PercevalHR intensities were measured from total photon counts. pHRed empirical lifetimes were averaged over a 9-ns window. The zero time offset for the averaging window was set as the time of peak intensity, which was estimated by fitting fluorescence decays to a bi-exponential function convoluted with the measured instrument response function. There was no difference in zero time offsets that were determined using a Gaussian or empirical instrument response function. Here fitting is only used to determine the zero time offset and averaging window, and the empirical mean lifetimes are reported because they provide a model-independent measurement. Two-photon absorption cross-sections were measured relative to a fluorescein standard (Invitrogen) according to Albota et al . [58] using the relationship: where σ 2 (λ) is the two-photon absorption cross-section, ϕ is the fluorescence quantum yield and F is the fluorescence signal. To use this simplified relationship [34] , we assume that collection efficiency, incident power and sample refractive indices are equal. Collection efficiency can be assumed to be equal because PercevalHR and fluorescein fluorescence emission spectra are nearly identical, and fluorescence signals were collected on the same instrument with little variation over repeats. Incident power was stable with an average coefficient of variation of 1.4±0.1% (mean±s.e.m.). The fluorescein standard was made to 3 μM in aqueous 0.1 M NaOH, and the fluorescein two-photon excitation cross-section ( σ 2,Fluorescein ( λ )· ϕ Fluorescein ) determined by Albota et al . [58] is available at the Cornell University Developmental Resource for Biophysical Imaging Optoelectronics website ( www.drbio.cornell.edu/cross_sections.html ). PercevalHR was made to 10 μM in buffer (100 mM MOPS, pH 7.4, 50 mM KCl, 5 mM NaCl) containing either 0.2 mM ATP and 10 mM MgCl 2 or 0.2 mM ADP and 1 mM EDTA. ATP and ADP solutions had negligible background fluorescence at these concentrations. Two-photon excitation fluorescence spectra were obtained between 780–1010, nm in 10 nm increments, and 5–9 spectra were averaged. The quantum yields of the ADP- and MgATP-loaded states of PercevalHR relative to fluorescein ( Supplementary Table S1 ) were used to estimate the two-photon absorption cross-sections. Live-cell fluorescence microscopy with two-photon excitation was performed on the same instrument. The laser was cycled between 840 and 950 nm wavelengths for two-photon excitation. HEK293 cells expressing PercevalHR and pHRed were continuously perfused by gravity flow with imaging solution (in mM: 140 NaCl, 2.5 KCl, 2 CaCl 2 , 1 MgCl 2 , 10 glucose, 10 HEPES (pH 7.4)) at room temperature. IAA was used at 1 mM final concentration added to the imaging solution, and NH 4 Cl was used at 15 mM final concentration for pH calibration [27] . Cells were imaged to obtain a baseline and then solution was switched to IAA. After the PercevalHR signal decreased and stabilized, a transient switch to NH 4 Cl for 2–5 min was made to obtain the pH calibration. Image analysis Images were acquired with iQ (Andor) or TILLvisION (Till Photonics) and analysed with ImageJ. Mean and s.d. background pixel intensities were measured for every field of view in every experiment. A background mask was created for each image frame using a minimum threshold of three times the s.d. of the background. Pixels containing fluorescent signal were selected by applying the background mask to intensity images, and pixel-by-pixel ratio images were calculated. Fluorescence ratios were calculated from the mean over a region of interest drawn around each analysed cell. How to cite this article: Tantama, M. et al . Imaging energy status in live cells with a fluorescent biosensor of the intracellular ATP-to-ADP ratio. Nat. Commun. 4:2550 doi: 10.1038/ncomms3550 (2013).